Stac3 is a component of the excitation–contraction coupling machinery and mutated in Native American myopathy Excitation–contraction coupling, the process that regulates contractions by skeletal muscles, transduces changes in membrane voltage by activating release of Ca 2+ from internal stores to initiate muscle contraction. Defects in excitation–contraction coupling are associated with muscle diseases. Here we identify Stac3 as a novel component of the excitation–contraction coupling machinery. Using a zebrafish genetic screen, we generate a locomotor mutation that is mapped to stac3 . We provide electrophysiological, Ca 2+ imaging, immunocytochemical and biochemical evidence that Stac3 participates in excitation–contraction coupling in muscles. Furthermore, we reveal that a mutation in human STAC3 is the genetic basis of the debilitating Native American myopathy (NAM). Analysis of NAM stac3 in zebrafish shows that the NAM mutation decreases excitation–contraction coupling. These findings enhance our understanding of both excitation–contraction coupling and the pathology of myopathies. Muscle contractions are initiated by depolarization of the voltage across the plasma membrane resulting from synaptic release at the neuromuscular junction (NMJ). Excitation–contraction (EC) coupling is responsible for transducing the shift in the membrane voltage to increase cytosolic levels of Ca 2+ that leads to contraction. Genetic defects in EC coupling components are associated with numerous congenital myopathies [1] that appear in infancy and are characterized by a variety of symptoms that include muscle weakness, difficulty with breathing and feeding, slower development, muscle cramps, stiffness and spasm, and in some cases susceptibility to malignant hyperthermia, which is an adverse reaction to general anaesthesia that can be fatal. Despite the debilitating nature of congenital myopathies, their pathology is for the most part poorly understood. Congenital myopathies are highly heterogenous, and the genetic basis of many disorders are unknown. In skeletal muscles, EC coupling occurs at triads. Triads are junctions of the transverse tubules that are infoldings of the sarcomembrane and the sarcoplasmic reticulum (SR), an internal Ca 2+ store. Changes in the membrane voltage of the transverse tubules are detected by the dihydropyridine receptor (DHPR), an L-type Ca 2+ channel located in the transverse tubule membrane at triads [2] , [3] , [4] , [5] . DHPR is composed of the principal α1s subunit also called Ca V 1.1 that contains the pore and several accessory subunits. Activated DHPR, in turn, is thought to directly activate ryanodine receptor 1 (RyR1) Ca 2+ release channels in the SR membrane side of the triadic junctions [6] , [7] , [8] , [9] . In mammalian skeletal muscles, the DHPR also conducts extracellular Ca 2+ to the cytosol but this is not required for EC coupling [10] . Interestingly, in teleost skeletal muscles EC coupling is similarly independent of Ca 2+ influx from the exterior and the DHPR appears to have evolved so that it no longer conducts Ca 2+ (ref. 11 ). Activation of RyR1 leads to release of Ca 2+ from the SR to the cytosol and subsequently to contraction mediated by the contractile machinery. EC coupling involves a complex of proteins localized to triads that include DHPR and RyR1. Although DHPR and RyR1 are well studied, the identity and roles of other components of the complex, how EC coupling is regulated and how the triadic molecular complex is established are poorly understood. Some of the other components of the triadic complex include FKBP12, triadin, junctin and calsequestrin. Triadin, junctin and calsequestrin are SR proteins that regulate RyR1 from the luminal side of SR [12] , [13] , [14] . FKBP12 is an immunophilin, an immunosuppressive drug-binding protein, that copurifies and co-immunoprecipitates with RyR1 in striated muscles [15] , and stabilize RyRs in their open state in vitro [16] . Two other cytosolic proteins that interact with EC components are SepN1 and calmodulin (CaM). SepN1 is a selenoprotein that co-immunoprecipitates with RyR1a and is associated with myopathy [17] and is required for formation of slow twitch muscles in zebrafish [18] . CaM can bind RyR and DHPR, and modify EC coupling [19] . Despite the identification of these factors, the mechanisms for how they regulate EC coupling is poorly understood. These analyses illustrate the complexity of the EC coupling complex and its regulation, and suggest that a forward genetic strategy might be useful for identification of novel components for EC coupling. Zebrafish have been useful for the analysis of a myriad of biological processes both because they are amenable to forward genetic screens and in vivo manipulations [20] , [21] . Pertinent to a genetic analysis of EC coupling, zebrafish muscles can also be analysed in vivo with electrophysiology and live imaging [22] , [23] . We took advantage of these features to identify a zebrafish mutation in which EC coupling was defective. The gene responsible for the mutant phenotype encoded for Stac3, a putative muscle-specific adaptor protein. Finally, we found that a missense mutation in human STAC3 is responsible for the debilitating, congenital Native American myopathy (NAM) [24] , [25] . The mi34 zebrafish mutant is defective in EC coupling To identify new genes involved in the regulation of EC coupling, a forward genetic screen in the zebrafish was performed to isolate motor behaviour mutants [26] , [27] , [28] , [29] , [30] . One mutation, mi34 , was autosomal recessive with mutants dying as larvae and exhibiting defective motor behaviours at early stages of development. Normally zebrafish embryos exhibited spontaneous slow coiling of the body starting at 17 h post fertilization (hpf), touch-induced escape contractions of the body at 22 hpf and touch-induced swimming by 28 hpf (ref. 31 ). Mutants were defective in all three motor behaviours with reduced amplitude of spontaneous coiling, decreased touch-induced escape contractions and ineffective swimming ( Supplementary Movies S1–6 ; Fig. 1a ). 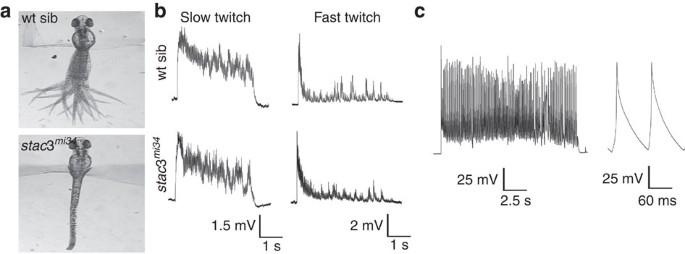Figure 1:mi34mutant zebrafish exhibit defective swimming but CNS output is normal. (a) Touch evoked swimming in wt but notstac3mi34embryos (48 hpf). Panels show superimposed frames (30 Hz) of swimming motion from wt sibling andstac3mi34embryos with heads embedded in agar. (b) Voltage recordings with 6-mM curare showing that touch-evoked synaptic responses of slow twitch (wt sib:n=5; mut:n=6) and fast twitch muscles (wt sib:n=6; mut:n=4) of wt sibling andstac3mi34mutants (48 hpf) are comparable. (c) Voltage recordings with no curare showing that mutant fast twitch muscles (48 hpf) respond to tactile stimulation with a burst of action potentials (n=8). Figure 1: mi34 mutant zebrafish exhibit defective swimming but CNS output is normal. ( a ) Touch evoked swimming in wt but not stac3 mi34 embryos (48 hpf). Panels show superimposed frames (30 Hz) of swimming motion from wt sibling and stac3 mi34 embryos with heads embedded in agar. ( b ) Voltage recordings with 6-mM curare showing that touch-evoked synaptic responses of slow twitch (wt sib: n =5; mut: n =6) and fast twitch muscles (wt sib: n =6; mut: n =4) of wt sibling and stac3 mi34 mutants (48 hpf) are comparable. ( c ) Voltage recordings with no curare showing that mutant fast twitch muscles (48 hpf) respond to tactile stimulation with a burst of action potentials ( n =8). Full size image Aberrant behaviour in mutants could be due to defects in the nervous system and/or skeletal muscles. If signalling within the nervous system were abnormal in mutants, then one would expect the output of motor neurons to muscles to be aberrant. To determine this, the synaptic response of muscles to tactile stimulation of the embryo was electrophysiologically recorded in vivo . Tactile stimulation initiated synaptic responses in both slow and fast twitch muscles in both wild-type (wt) sibling and mutant embryos. The evoked responses were comparable in amplitude, duration and frequency, when measured with a low concentration of curare (see Methods) used to minimize muscle contraction ( Fig. 1b ; Supplementary Fig. S1 ). To see if the mutant muscles would generate action potentials in response to synaptic input, we examine muscle responses following sensory stimulation without curare, which was possible because contraction by mutant muscles is minimal. These recordings showed that mutant fast twitch muscles do respond with a burst of overshooting action potentials ( Fig. 1c ). Furthermore, there were no obvious differences in the distribution of motor neuron terminals and muscle acetylcholine receptors (AChRs) between wt sibs and mutants when assayed with an antibody against SV2, a synaptic vesicle protein, and α-bungarotoxin that specifically binds AChRs ( Supplementary Fig. S2 ). Thus, the nervous system and NMJ between wt and mutants is comparable and mutant muscles can initiate bursts of action potentials in response to synaptic input. Although we cannot rule of subtle changes, the severity of the behavioural phenotype is consistent with the mutation causing a defect in the muscle response to electrophysiological activation. Activation of the NMJ leads to depolarization of the muscle membrane potential that in turn initiates muscle contraction. To examine how the mutation affects the relationship between muscle voltage and contraction, the membrane voltage of skeletal muscles was depolarized to various values and the amount muscles contracted was measured. Mutant muscles contracted much less than wt sib muscles at depolarized membrane potentials ( Supplementary Fig. S3 ). The decreased contraction to depolarizations could be due to a defect in EC coupling or a defect in the contractile machinery. However, the fact that mutant and wt sib muscles contracted similarly when exposed to caffeine, an agonist of RyRs, ( Supplementary Fig. S4 ) suggested that the contractile machinery was intact in mutants and that the store of Ca 2+ in the SR was not grossly perturbed. Corroborating this finding, mutant muscles exhibited no obvious morphological defects early in the development with apparent normal distribution of contractile proteins and other muscle proteins ( Supplementary Fig. S4 ). Furthermore, myofibers appeared normal in electron micrographs of larval skeletal muscles in mi34 mutants ( Fig. 2a ). These findings pointed to a defect in EC coupling in mutant muscles. 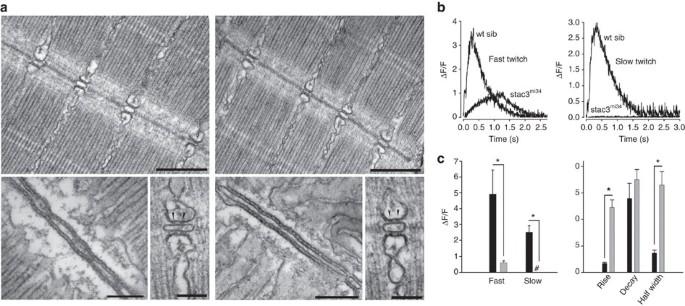Figure 2: EC coupling is defective inmi34mutant zebrafish embryos. Electron micrographs showing that the ultrastructure of myofibrils and triadic junctions are comparable between the muscles of 4 days post fertilization (dpf) wt sibling (a, left) andmi34mutants (a, right). Top: longitudinal sections showing several myofibrils and triads sectioned at right angle to the T tubule long axis. Scale: 500 nm. Bottom: at left a section tangent to the triad, showing one of the two long rows of feet (RyR) that occupy the junctional gap. Scale: 250 nm. Bottom: at right a section transverse to the triad axis showing two feet (arrowheads) in the junctional gap of the triad. Scale: 100 nm. (b) Ca2+transients recorded from GCaMP3-expressing fast and slow twitch fibres are significantly decreased and slower in 48 hpfstac3mi34mutants. (c) Left: quantification of peak Ca2+release with black and grey bars representing wt sib (fast,n=5; slow,n=5) andstac3mi34(fast,n=9; slow,n=7) fibres, respectively. #Denotes that peak Ca2+was 0. Right: quantification of Ca2+transient kinetics in fast fibres with black and grey bars representing wt sib andstac3mi34, respectively. Half width denotes the duration the transient is >50% of peak value. Error bars represent s.e.m.’s. Asterisks signifiesP<0.01,t-test. Figure 2: EC coupling is defective in mi34 mutant zebrafish embryos. Electron micrographs showing that the ultrastructure of myofibrils and triadic junctions are comparable between the muscles of 4 days post fertilization (dpf) wt sibling ( a , left) and mi34 mutants ( a , right). Top: longitudinal sections showing several myofibrils and triads sectioned at right angle to the T tubule long axis. Scale: 500 nm. Bottom: at left a section tangent to the triad, showing one of the two long rows of feet (RyR) that occupy the junctional gap. Scale: 250 nm. Bottom: at right a section transverse to the triad axis showing two feet (arrowheads) in the junctional gap of the triad. Scale: 100 nm. ( b ) Ca 2+ transients recorded from GCaMP3-expressing fast and slow twitch fibres are significantly decreased and slower in 48 hpf stac3 mi34 mutants. ( c ) Left: quantification of peak Ca 2+ release with black and grey bars representing wt sib (fast, n =5; slow, n =5) and stac3 mi34 (fast, n =9; slow, n =7) fibres, respectively. #Denotes that peak Ca 2+ was 0. Right: quantification of Ca 2+ transient kinetics in fast fibres with black and grey bars representing wt sib and stac3 mi34 , respectively. Half width denotes the duration the transient is >50% of peak value. Error bars represent s.e.m.’s. Asterisks signifies P <0.01, t -test. Full size image The hallmark of EC coupling is the release of Ca 2+ from the SR to the cytosol. EC coupling was directly examined in vivo by imaging Ca 2+ transients in skeletal myofibers, expressing the GCaMP3 Ca 2+ indicator [32] during swimming. Swimming was evoked by application of NMDA, which activated the swimming network in the central nervous system [28] . Ca 2+ transients were greatly reduced in both mutant slow and fast twitch fibres ( Fig. 2b ). Thus, EC coupling in skeletal muscles was defective in the mi34 mutants. As EC coupling takes place at triads, reduced EC coupling in mutants could be due to abnormal formation of triads. However, longitudinal sections examined with transmission electron microscopy showed that there were triads at every intermyofibrillar junction with triads exhibiting comparable anatomy including two rows of feet in wt sib and mutant muscles ( Fig. 2a ). Although we cannot rule out a quantitative change in triadic anatomy, these data showed that the decrease in EC coupling in mutant muscles was not due to any obvious defect in triad anatomy. stac3 is the basis for the mi34 phenotype A combination of meiotic mapping and analysis of zebrafish genome resources identified the gene responsible for the mi34 phenotype as stac3 ( Supplementary Fig. S5 ; for details see Methods), a gene similar to murine stac that encodes an adaptor-like protein of unknown function [33] . stac3 encodes for a putative 334 residue soluble protein with an N-terminal cysteine-rich domain (CRD) similar to the C1 domain found in Ca-dependent protein kinase and two SH3 domains ( Fig. 3a ). The mutant allele carried a point mutation that disrupted a splice donor site that led to the inclusion of intron 4 and a premature stop codon in the transcript. The mutation in stac3 predicted a protein that was truncated within the N-terminal CRD, suggesting that the stac3 mi34 mutation was functionally null. Western blotting with an antibody generated against Stac3 that recognized a fragment of Stac3 consisting of the residues 1–63 (see Methods) revealed an ~49 kDa protein in wt embryos but no protein in mutants ( Fig. 3b ), suggesting that a truncated protein was not synthesized in mutants. In situ hybridization showed that skeletal muscles selectively expressed stac3 during embryogenesis ( Supplementary Fig. S6 ). Labelling with anti-Stac3 confirmed that Stac3 was specifically expressed by skeletal muscles and revealed that Stac3 co-localized with the DHPR α1 and presumably RyR1 at muscle triads in wt but was not expressed in mutant embryos ( Fig. 3c ). These findings suggested that a mutation in stac3 was responsible for defective EC coupling and that Stac3 was a component of the triadic molecular complex. 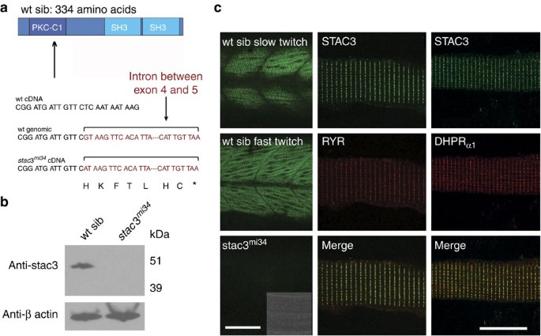Figure 3: The muscle-specific genestac3underlies themi34phenotype. (a) Diagram of the predicted wt Stac3 protein (top). Arrow denotes location of the stop codon. DNA sequence of corresponding regions of wt cDNA, wt genomic DNA andstac3mi34cDNA showing that a missense mutation in a splice donor site lead to the inclusion of the intron (bracket) and stop codon (asterisk) in the mutant cDNA. (b) Stac3 protein appears not to be synthesized in mutants. Western blot of showing that anti-Stac3 labels a band from wt but not mutant embryos at 48 hpf. β-Actin was the loading control. (c) Stac3 co-localizes with RyR and DHPRα1in the skeletal muscles. Left, side view of the trunk of 48 hpf embryos labelled with anti-Stac3 showing that both fast twitch and slow twitch express Stac3 in wt but not mutant embryos. Scale: 60 μm. Inset shows the brightfield image of the trunk of the mutant. Right, dissociated 48 hpf wt muscle fibres labelled with anti-Stac3 and anti-RyR or anti-DHPRα1showing that Stac3 co-localizes with RyR and DHPRα1. Scale: 10 μm. Figure 3: The muscle-specific gene stac3 underlies the mi34 phenotype. ( a ) Diagram of the predicted wt Stac3 protein (top). Arrow denotes location of the stop codon. DNA sequence of corresponding regions of wt cDNA, wt genomic DNA and stac3 mi34 cDNA showing that a missense mutation in a splice donor site lead to the inclusion of the intron (bracket) and stop codon (asterisk) in the mutant cDNA. ( b ) Stac3 protein appears not to be synthesized in mutants. Western blot of showing that anti-Stac3 labels a band from wt but not mutant embryos at 48 hpf. β-Actin was the loading control. ( c ) Stac3 co-localizes with RyR and DHPR α1 in the skeletal muscles. Left, side view of the trunk of 48 hpf embryos labelled with anti-Stac3 showing that both fast twitch and slow twitch express Stac3 in wt but not mutant embryos. Scale: 60 μm. Inset shows the brightfield image of the trunk of the mutant. Right, dissociated 48 hpf wt muscle fibres labelled with anti-Stac3 and anti-RyR or anti-DHPR α1 showing that Stac3 co-localizes with RyR and DHPR α1 . Scale: 10 μm. Full size image The molecular identity of the mutation was confirmed by mutant rescue experiments. Induced expression of hsp70:stac3 wt -egfp in mutant muscles rescued the behavioural phenotype and triadic localization of Stac3, whereas induced expression of hsp70:stac3 mi34 -egfp did not ( Fig. 4a ). Furthermore, Ca 2+ imaging of mutant muscles coexpressing stac3 wt -mCherry and GCaMP3 showed that wt Stac3 could restore Ca 2+ muscle transients in mutant embryos ( Fig. 4b ). Given that Stac3 may be an adaptor protein and co-localizes with DHPR α1 and RyR1, we examined whether Stac3 may be part of the triadic molecular complex. Indeed co-immunoprecipations with antibodies against pan-RyR and DHPR α1 both pulled down Stac3 from wt adult muscles ( Fig. 5 ), indicating that Stac3 is part of the DHPR/RyR1 complex found at triads. This was confirmed by generating a transgenic line of zebrafish (α -actin:stac3 wt -egfp ) that expressed Stac3-EGFP in the skeletal muscles and by using anti-GFP to immunoprecipitate Stac3-EGFP from lysates of skeletal muscle of adult transgenic zebrafish. Mass spectrometry-based protein identification found that DHPR α1s , DHPR α2δ1 , DHPR β1 , RyR1 and RyR3 immunoprecipitated with Stac3-EGFP ( Supplementary Table S1 ). Thus, Stac3 is a component of the triadic complex that is required for EC coupling in skeletal muscles. 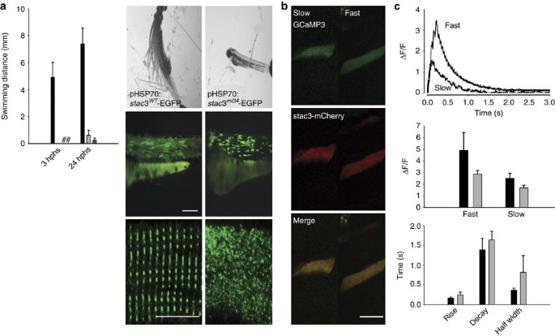Figure 4: Expression of wt Stac3 in muscles rescues thestac3mi34phenotype. (a) Left, histogram showing that mutant embryos expressing heat-induciblestac3wt-egfp(black,n=32) but notstac3mi34-egfp(light grey,n=4) nor uninjected mutant embryos (dark grey,n=10) exhibited touch-evoked swimming at both 3 h post heat shock (hphs) and 24 hphs. #Denotes no swimming. Right panels, superimposed frames (30 Hz, 1 s) (top) show that mutant embryos expressingstac3wtbut notstac3mi34swim in response to touch, although both are similarly expressed by muscles (middle, scale: 180 μm). In dissociated mutant muscles Stac3wt-EGFP localizes to the triads but not Stac3mi34-EGFP (bottom, scale: 10 μm). (b)In vivoexpression of Stac3wt-mCherry by mutant muscle fibres rescues Ca2+transients. Left panels,stac3mi34mutant slow and fast twitch fibres coexpressingα-actin-driven GCaMP3 and heat-induced Stac3wt-mCherry. The triadic localization of Stac3wt-mCherry cannot be seen due to the low resolution of the resonance scans used to detect the fluorescent proteins. (c) Top, Ca2+transients from mutant fast and slow fibres coexpressing Stac3wt-mCherry and GCaMP3. Middle, histogram showing that peak Ca2+release is comparable between wt (black) fast (n=5) and slow (n=5) fibres, and rescued mutant (grey) fast (n=6) and slow (n=2) fibres. Bottom, histogram showing that the kinetics of Ca2+transients from wt (black) and rescued mutant (grey) fast twitch fibres are comparable. Error bars represent s.e.m.’s. Figure 4: Expression of wt Stac3 in muscles rescues the stac3 mi34 phenotype. ( a ) Left, histogram showing that mutant embryos expressing heat-inducible stac3 wt -egfp (black, n =32) but not stac3 mi34 -egfp (light grey, n =4) nor uninjected mutant embryos (dark grey, n =10) exhibited touch-evoked swimming at both 3 h post heat shock (hphs) and 24 hphs. #Denotes no swimming. Right panels, superimposed frames (30 Hz, 1 s) (top) show that mutant embryos expressing stac3 wt but not stac3 mi34 swim in response to touch, although both are similarly expressed by muscles (middle, scale: 180 μm). In dissociated mutant muscles Stac3 wt -EGFP localizes to the triads but not Stac3 mi34 -EGFP (bottom, scale: 10 μm). ( b ) In vivo expression of Stac3 wt -mCherry by mutant muscle fibres rescues Ca 2+ transients. Left panels, stac3 mi34 mutant slow and fast twitch fibres coexpressing α-actin -driven GCaMP3 and heat-induced Stac3 wt -mCherry. The triadic localization of Stac3 wt -mCherry cannot be seen due to the low resolution of the resonance scans used to detect the fluorescent proteins. ( c ) Top, Ca 2+ transients from mutant fast and slow fibres coexpressing Stac3 wt -mCherry and GCaMP3. Middle, histogram showing that peak Ca 2+ release is comparable between wt (black) fast ( n =5) and slow ( n =5) fibres, and rescued mutant (grey) fast ( n =6) and slow ( n =2) fibres. Bottom, histogram showing that the kinetics of Ca 2+ transients from wt (black) and rescued mutant (grey) fast twitch fibres are comparable. Error bars represent s.e.m.’s. 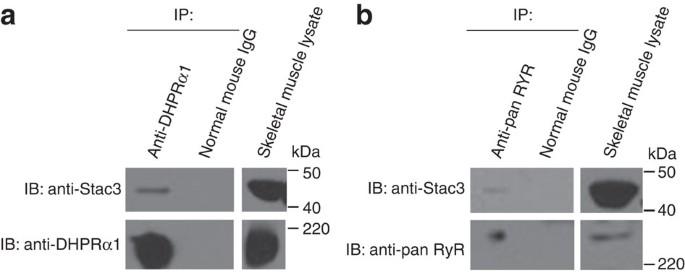Figure 5: Stac3 forms a molecular complex with DHPR and RyR. (a) Immunoblots (IB) showing that immunoprecipitation (IP) with anti-DHPRα1but not mouse IgG pulls down DHPRα1and Stac3 from adult skeletal muscle lysate (n=3). Skeletal muscle lysate lane is a immunoblot showing Stac3 and DHPRα1are expressed by muscles. (b) Immunoblots showing that immunoprecipitation with anti-pan-RyR but not mouse IgG pulls down RyR and Stac3 from adult skeletal muscle lysate (n=3). Skeletal muscle lysate lane is a immunoblot, showing Stac3 and RyR are expressed by the muscles. Full size image Figure 5: Stac3 forms a molecular complex with DHPR and RyR. ( a ) Immunoblots (IB) showing that immunoprecipitation (IP) with anti-DHPR α1 but not mouse IgG pulls down DHPR α1 and Stac3 from adult skeletal muscle lysate ( n =3). Skeletal muscle lysate lane is a immunoblot showing Stac3 and DHPR α1 are expressed by muscles. ( b ) Immunoblots showing that immunoprecipitation with anti-pan-RyR but not mouse IgG pulls down RyR and Stac3 from adult skeletal muscle lysate ( n =3). Skeletal muscle lysate lane is a immunoblot, showing Stac3 and RyR are expressed by the muscles. Full size image Although motor behaviours are greatly diminished in stac3 mi34 mutants, they were not immotile. One possible reason for this might be the existence and action of Stac3 derived from maternally deposited stac3 mRNA. In fact, RT-PCR (PCR with reverse transcription) from 2hpf embryos (before zygotic expression [34] ) found that stac3 was maternally expressed ( Fig. 6a ). To see whether the residual activity of skeletal muscles in stac3 mi34 mutants was due to Stac3 translated from maternal mRNA, we knocked down Stac3 by injecting a translation-blocking antisense Morpholino oligonucleotide (MO) against stac3 message into embryos from crosses between heterozygous carriers. Anti-Stac3 labelling showed that stac3 antisense MO-injected embryos did not express Stac3 in the skeletal muscles ( Fig. 6b ), confirming that the MO was effective. At 48 hpf wt embryos normally respond to tactile stimulation by swimming away. As expected from a cross between heterozygous carriers ~75% of the progeny injected with control MO responded to touch with swimming whereas 25% responded by slight muscle contractions (shivering) that failed to move the embryos effectively or were totally immotile ( Fig. 6c ), indicative of the mutant phenotype. In antisense MO-injected embryos, however, there was a significant increase in embryos that were either immotile or shivered and decrease in embryos that swam compared with control progeny. Significantly the proportion of immotile embryos increased from ~5% of control MO-injected progeny to almost 40% of antisense MO-injected progeny. Furthermore, the morphant phenotype was rescued by coinjecting an expression plasmid for stac3 wt along with the antisense MO, demonstrating that the increased defective motility observed was not due to an off-target effect of the antisense MO, but rather a specific knockdown of maternal stac3 . This suggests that elimination of both maternal and zygotic Stac3 results in immotility. 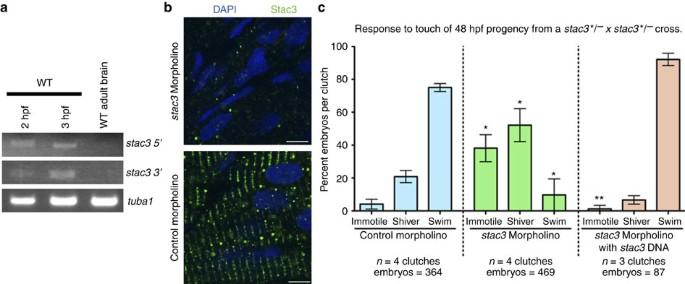Figure 6:stac3mRNA is maternally expressed. (a) RT-PCR from 2 and 3 hpf embryos showing thatstac3mRNA is maternally expressed. Midblastula transition starts at 3 hpf.stac3mRNA is not expressed in the adult brain.tuba1,a house-keeping gene that is maternally expressed, serves as a positive control andstac3in the adult brain as a negative control.stac35′ and 3′ refer to primers used for amplifying either 5′ or 3′ fragments ofstac3fromstac3cDNA (see Methods). (b) Micrographs showing anti-Stac3 labelled embryos (48 hpf) that had been injected withstac3antisense MO (top) but not control MO (bottom) exhibit little to no Stac3. Muscle nuclei are labelled with 4′,6-diamidino-2-phenylindole (DAPI; blue). Scale: 5 μm. (c) Knocking down Stac3 in 48 hpf embryos significantly increases the proportion of progeny from a cross betweenstac3mi34heterozygous carriers that are immotile or shiver and decreases those that swim in response to touch. *Denotes that the percentage ofstac3MO-injected progeny that were immotile or shivered was greater than control MO-injected progeny (respectively,P<0.001 andP<0.01;t-test); percentage ofstac3MO-injected progeny that swam was less than control MO-injected progeny (P<0.001,t-test). **Denotes that coinjection of an expression plasmid forstac3wtwithstac3antisense MO decreases immotility and restores swimming in a great majority of progeny. Percentage ofstac3MO+expression plasmid forstac3wt-injected progeny that were immotile was much less thanstac3MO alone progeny (P<0.001,t-test). Error bars represent s.e.m.’s. Figure 6: stac3 mRNA is maternally expressed. ( a ) RT-PCR from 2 and 3 hpf embryos showing that stac3 mRNA is maternally expressed. Midblastula transition starts at 3 hpf. stac3 mRNA is not expressed in the adult brain. tuba1, a house-keeping gene that is maternally expressed, serves as a positive control and stac3 in the adult brain as a negative control. stac3 5′ and 3′ refer to primers used for amplifying either 5′ or 3′ fragments of stac3 from stac3 cDNA (see Methods). ( b ) Micrographs showing anti-Stac3 labelled embryos (48 hpf) that had been injected with stac3 antisense MO (top) but not control MO (bottom) exhibit little to no Stac3. Muscle nuclei are labelled with 4′,6-diamidino-2-phenylindole (DAPI; blue). Scale: 5 μm. ( c ) Knocking down Stac3 in 48 hpf embryos significantly increases the proportion of progeny from a cross between stac3 mi34 heterozygous carriers that are immotile or shiver and decreases those that swim in response to touch. *Denotes that the percentage of stac3 MO-injected progeny that were immotile or shivered was greater than control MO-injected progeny (respectively, P <0.001 and P <0.01; t -test); percentage of stac3 MO-injected progeny that swam was less than control MO-injected progeny ( P <0.001, t -test). **Denotes that coinjection of an expression plasmid for stac3 wt with stac3 antisense MO decreases immotility and restores swimming in a great majority of progeny. Percentage of stac3 MO+expression plasmid for stac3 wt -injected progeny that were immotile was much less than stac3 MO alone progeny ( P <0.001, t -test). Error bars represent s.e.m.’s. Full size image A mutation in human STAC3 causes a congenital myopathy The loss of Stac3 resulted in a progressive breakdown of myofibers during larval stages with apparent swollen SR observed by 7 days post fertilization ( Supplementary Fig. S7 ). Given the myopathic features of mutants, we explored whether stac3 mutations might cause congenital human myopathies. Human STAC3 mapped to chromosome 12q13-14, and its specific location was within the previously defined genetic locus for the congenital NAM (refs 24 , 25 ). NAM is an autosomal recessive disorder found within the Lumbee Native American population of North Carolina that was characterized by a constellation of clinical features, including congenital onset of muscle weakness, susceptibility to malignant hyperthermia, multiple joint contractures and dysmorphic facial features including ptosis. Patient muscle biopsies revealed a non-specific myopathic pattern. Furthermore, 36% of afflicted individuals die by the age of 18. The genetic basis of NAM remained unsolved, though the presence of susceptibility to malignant hyperthermia as a clinical feature suggested a defect in a component of the EC coupling apparatus. To see whether a mutation in STAC3 was the basis for NAM, STAC3 -coding regions were sequenced in a cohort of five NAM families that included 5 affected and 13 unaffected individuals. As expected for an autosomal recessive disorder, all affected individuals were homozygous for a G>C missense mutation of base pair 1,046 in exon 10 of the STAC3 gene (Ensembl transcript ID ENST00000332782), while all obligate carriers were heterozygous. This mutation resulted in a tryptophan (W) to serine (S) substitution at amino acid 284 in the first SH3 domain ( Fig. 7 ). The sequence change perfectly segregated with the NAM phenotype, and was neither found in an additional three unaffected, unrelated Lumbee individuals ( Supplementary Fig. S8 ), nor in 113 Caucasian control individuals. In addition, STAC3 has been sequenced as part of the 1,000 genome project, and this mutation has not been detected. This pattern of inheritance suggested that STAC3 was the basis for the congenital myopathy. 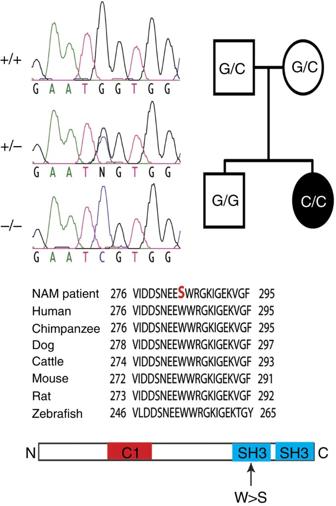Figure 7: Missense mutation in humanSTAC3causes NAM. Left top, sequence chromatographs of corresponding exonic region of theSTAC3gene of individuals that were +/+, +/− and −/− for the NAM locus showing the G>C missense mutation in thestac3gene. N denotes the G/C heterozygous nucleotide. Right top, pedigree of an individual exhibiting NAM (black) and homozygous for the missense mutation (C/C). Unaffected parents were carriers for the mutation (G/C) and the unaffected sibling was homozygous for the wt nucleotide (G/G). Middle, alignment of the corresponding region of Stac3 containing NAM mutation showing that the missense mutation results in a W>S substitution in NAM individuals and that this W is completely conserved between various mammals and zebrafish. Bottom, diagram showing that the missense mutation in Stac3NAMis located in a SH3 domain. Figure 7: Missense mutation in human STAC3 causes NAM. Left top, sequence chromatographs of corresponding exonic region of the STAC3 gene of individuals that were +/+, +/− and −/− for the NAM locus showing the G>C missense mutation in the stac3 gene. N denotes the G/C heterozygous nucleotide. Right top, pedigree of an individual exhibiting NAM (black) and homozygous for the missense mutation (C/C). Unaffected parents were carriers for the mutation (G/C) and the unaffected sibling was homozygous for the wt nucleotide (G/G). Middle, alignment of the corresponding region of Stac3 containing NAM mutation showing that the missense mutation results in a W>S substitution in NAM individuals and that this W is completely conserved between various mammals and zebrafish. Bottom, diagram showing that the missense mutation in Stac3 NAM is located in a SH3 domain. Full size image Next the functional consequences of the W284S mutation was investigated in the zebrafish model system. The analogous W>S substitution was encoded in zebrafish stac3 ( hsp70:stac3 NAM -egfp ) and expressed in stac3 mi34 -null mutant muscles to assay for phenotypic rescue. Unlike stac3 wt -egfp , expression of stac3 NAM -egfp failed to rescue touch-induced swimming, although some Stac3 NAM localized to triads ( Fig. 8a ). Furthermore, Ca 2+ imaging of mutant fast but not slow twitch muscles expressing stac3 NAM -mCherry and GCaMP3 exhibited Ca 2+ transients that were decreased compared with mutant muscles expressing stac3 wt -mCherry and GCaMP3 ( Figs 4b and 8b ). Presumably the mosaic expression of a partially effective allele was insufficient to result in behavioural rescue. Decreased Ca 2+ transients in fast twitch but not slow twitch muscles expressing stac3 NAM predicts defective swimming, as by 48 hpf swimming is dependent on fast twitch muscle contractions and independent of slow twitch contractions [35] . Additionally, expression of wt human STAC3 in mutant zebrafish muscles rescued the motor phenotype ( Supplementary Fig. S9 ). Thus, the NAM mutation appeared to diminish EC coupling in fast twitch muscles and was causative for the congenital myopathy. 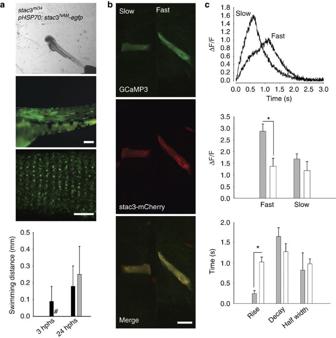Figure 8: Thestac3NAMallele decreases EC coupling. (a) Expression of Stac3NAMby muscle fibres instac3mi34embryos does not rescue touch-evoked swimming. Superimposed frames (30 Hz) showing that a heat-induced mutant embryo previously injected withpHSP70:stacNAM-egfpdoes not swim following tactile stimulation (top), despite expression of zebrafish Stac3NAM-EGFP in myotomes and triadic localization of zebrafish Stac3NAM-EGFP (middle, scale bars: 180 and 10 μm). Histograms (bottom) quantify the comparable lack of touch-evoked swimming ofstac3mi34mutants expressing the NAM allele (black) and uninjected mutants (grey) both 3 and 24 h post heat shock (hphs). Note the difference in scale of theyaxis from that inFig. 4athat shows swimming in mutant rescued embryos. #Denotes zero movement. (b) Expression of Stac3NAMby muscle fibres instac3mi34embryos partially rescues Ca2+transientsin vivo. Examples ofstac3mi34mutant slow and fast twitch fibres coexpressingα-actin-driven GCaMP3 andhsp70-regulated zebrafish Stac3NAM-mCherry. The triadic localization of Stac3wt-mCherry cannot be seen due to the low resolution of the resonance scans used to detect the fluorescent proteins. (c) Top, Ca2+transients from mutant fast and slow fibres coexpressing Stac3NAM-mCherry and GCaMP3. Middle, histogram showing that peak Ca2+release is decreased between mutant fast fibres expressingstac3wt(grey,n=6) andstac3NAM(white,n=6). Peak Ca2+was not different for mutant slow twitch fibres (wt,n=2; NAM allele,n=2). Bottom, histogram showing the kinetics of Ca2+transients of mutant fast fibres expressingstac3wt(grey,n=5) andstac3NAM(white,n=9). Asterisk signifiesP<0.01,t-test. Error bars represent s.e.m.’s. Figure 8: The stac3 NAM allele decreases EC coupling. ( a ) Expression of Stac3 NAM by muscle fibres in stac3 mi34 embryos does not rescue touch-evoked swimming. Superimposed frames (30 Hz) showing that a heat-induced mutant embryo previously injected with pHSP70:stac NAM -egfp does not swim following tactile stimulation (top), despite expression of zebrafish Stac3 NAM -EGFP in myotomes and triadic localization of zebrafish Stac3 NAM -EGFP (middle, scale bars: 180 and 10 μm). Histograms (bottom) quantify the comparable lack of touch-evoked swimming of stac3 mi34 mutants expressing the NAM allele (black) and uninjected mutants (grey) both 3 and 24 h post heat shock (hphs). Note the difference in scale of the y axis from that in Fig. 4a that shows swimming in mutant rescued embryos. #Denotes zero movement. ( b ) Expression of Stac3 NAM by muscle fibres in stac3 mi34 embryos partially rescues Ca 2+ transients in vivo . Examples of stac3 mi34 mutant slow and fast twitch fibres coexpressing α-actin -driven GCaMP3 and hsp70 -regulated zebrafish Stac3 NAM -mCherry. The triadic localization of Stac3 wt -mCherry cannot be seen due to the low resolution of the resonance scans used to detect the fluorescent proteins. ( c ) Top, Ca 2+ transients from mutant fast and slow fibres coexpressing Stac3 NAM -mCherry and GCaMP3. Middle, histogram showing that peak Ca 2+ release is decreased between mutant fast fibres expressing stac3 wt (grey, n =6) and stac3 NAM (white, n =6). Peak Ca 2+ was not different for mutant slow twitch fibres (wt, n =2; NAM allele, n =2). Bottom, histogram showing the kinetics of Ca 2+ transients of mutant fast fibres expressing stac3 wt (grey, n =5) and stac3 NAM (white, n =9). Asterisk signifies P <0.01, t -test. Error bars represent s.e.m.’s. Full size image This study identified Stac3 as a novel component of EC coupling in skeletal muscles, and a mutation in STAC3 as the cause for NAM. A recent study suggested that MO-mediated knockdown of stac3 in zebrafish embryos resulted in defective myofibrillar formation in skeletal muscles [36] , but we found that myofibrils in embryonic and larval zebrafish were comparable between wt sibs and stac3 mutants. This discrepancy might be due to the maternal wt stac3 transcript found in stac3 nulls, which could have been sufficient for normal myofibrillar formation in mutants. In principle, Stac3 could participate in EC coupling via a variety of mechanisms. One possibility is that Stac3 might modulate the channel properties of DHPR and/or RyR1. The triadic localization of Stac3 and biochemical demonstration that Stac3 is part of the DHPR/RyR1 complex are consistent with this possibility. Regulation of DHPR or RyR1 channel properties by other triadic components include modulation of the properties of DHPR by RyR1 and of RyR1 by FKBP12. In murine RyR1-deficient myotubes, the complement of DHPR on the muscle membrane is normal, but the DHPRs pass much less Ca 2+ than normal [37] . The immunophilin, FKBP12, copurifies with RyR, and anti-FKBP12 can pull down RyR in striated muscles [14] . When RyRs were examined with single channel recordings, FKBP12 was found to optimize channel function [15] . The β-subunits of voltage-dependent Ca channels are also known to regulate properties of a variety of Ca channels [38] . It is possible that Stac3 could interact with the β 1a -subunit to regulate DHPR channel properties in the skeletal muscles. Another possibility is that Stac3 may regulate the precise organization of DHPRs and RyR1s at triadic junctions of the t-tubules and SR. At triads, DHPRs and RyR1s are organized in a precise manner with DHPRs arranged in geometrically arranged groups of four called tetrads, with each tetrad apposed to every other RyR1 homotetramer [39] . The β 1a -subunit of DHPR also appears to be critical for this, as β 1a is required for the formation of DHPRs into tetrads [23] . Stac3 might also regulate the amount of DHPR and/or RyR1 at triads, perhaps by modulating protein trafficking and/or stability of DHPR and/or RyR1. An example of a factor that may be important for trafficking or stability of DHPRs is REM, a member of the RGK GTP-binding protein family. REM can bind β-subunits of voltage-dependent Ca 2+ channels, when expressed heterologously, and overexpression of REM inhibits L-type Ca 2+ channels in C2C12 cells [40] and skeletal muscles due to a decrease of DHPR in the muscle membrane [41] via dynamin-dependent endocytosis [42] . Although the loss-of-function phenotype for REM is not known, these results suggest that REM inhibits localization of DHPRs in triads either by decreasing processing of the channels into triadic junctions or by increasing the removal of the channel from triads. Interestingly the DHPR β1 subunit regulates the levels of plasma membrane DHPR α1c (Ca V 1.2) that is expressed by cardiac muscle cells and neurons by inhibiting the degradation of these channels via endoplasmic reticulum-associated protein degradation [43] . Examination of the amount of DHPR and RyR1 at triads in stac3 mutants versus wt muscles should clarify whether Stac3 controls the levels of these key components in skeletal muscles. Furthermore, it should be possible to investigate whether Stac3 regulates protein trafficking of key components of EC coupling using various transgenics combined with live-imaging strategies in zebrafish to directly examine fluorescently labelled EC components, as they are trafficked from the ER to triads and are endocytotically removed from the triads. Furthermore, the availability of mutants deficient for DHPR (refs 23 , 29 ) and RyR1 (ref. 30 ), in addition to the stac3 mi34 mutant, should be invaluable for mechanistic analysis of Stac3 for EC coupling. The NAM mutation converted W284 to S in the first SH3 domain of Stac3. Interestingly, an analysis of binding specificities of SH3 domains using a generic structure-based model found that this W, which is in the loop region of the SH3 domain and is highly conserved across SH3 domains, is one of the most important residues for binding specificity [44] . Our finding that expression of Stac3 NAM in Stac3-null zebrafish leads to decreased EC coupling suggests that interactions of the first SH3 domain in Stac3 is important for normal EC coupling. In fact, components of the triadic molecular complex including DHPR α1s , DHPR β1a and RyR1 contain numerous SH3-binding sequences in their predicted cytoplasmic portions. Thus, it would be interesting to see whether Stac3 might interact with triadic components such as DHPR and/or RyR1 via the Stac3 SH3 domain and whether such an interaction is necessary for normal EC coupling. Interestingly, the structure-based model also identified three other residues found in human Stac3 (Y255, E283 and N299) that also significantly affected binding specificity [44] . The roles of these residues for EC coupling could be examined by expressing appropriately mutagenized Stac3 in the zebrafish stac3 nulls. Genetic and physiological approaches should also be useful for the generation of transgenic lines of stac3 NAM mutant zebrafish to delineate the pathology of NAM and for identifying potential therapeutic agents. This is particularly relevant, given the increasing recognition of mutations in genes associated with EC coupling in a growing range of human muscle diseases. In addition, STAC3 is an attractive candidate for the genetic basis of currently undefined congenital myopathies, particularly those associated with susceptibility to malignant hyperthermia and/or those with phenotypes similar to those of patients with RYR1 or DHPR mutations. Animals and behavioural analysis Zebrafish were bred and maintained according to approved guidelines of the University Committee on Use and Care of Animals at the University of Michigan. The stac3 mi34 mutation was isolated from a mutagenesis screen using procedures previously reported [19] , [20] . Embryonic behaviours were video recorded with a CCD camera mounted on a stereomicroscope and analysed with ImageJ. In some cases, the heads of embryos were embedded in low melting temperature agar with the trunk and tail free to move. Where indicated data were analysed by t -tests. Electrophysiology Previously published protocols were followed to electrophysiologically record from zebrafish embryonic muscles [21] . For recordings embryos were partially curarized (6 μM d-tubocurarine). Recordings of muscle responses to touch were made with patch electrodes (3–10 MΩ) filled with solution containing 105 mM K gluconate, 16 mM KCl, 2 mM MgCl 2 , 10 mM Hepes, 10 mM EGTA and 4 mM Na 3 ATP at 273 mOsm and pH 7.2 and extracellular Evans solution (134 mM NaCl, 2.9 mM KCl, 2.1 mM CaCl 2 , 1.2 mM MgCl 2 , 10 mM glucose and 10 mM Hepes at 290 mOsm and pH 7.8) using an Axopatch 200B amplifier (Axon Instruments), low-pass filtered at 5 kHz and sampled at 1 kHz. Mechanosensory stimulation was delivered by ejecting bath solution from a pipette using a Picospritzer. Voltage dependence of contraction was performed in a similar manner except embryos were exposed to 50 μM d-tubocurarine, voltage steps delivered to muscle via voltage clamp and muscle contractions video recorded at 60 Hz. Muscle contractions to caffeine applied by a Picospritzer (10 psi, 1 s) of dissected embryos were video recorded and measured. Ca 2+ imaging One-cell stage embryos were injected with a plasmid using α-actin promoter [29] ( α-actin:GCaMP3 ) resulting in embryos that mosaically expressed α-actin:GCaMP3 within skeletal muscle. Forty-eight hours post fertilization embryos were genotyped by behaviour. Before imaging, tricaine was removed and embryos allowed to recover in Evans for 10 min and treated with 200 μM N-benzyl-p-toluene sulphonamide to inhibit contraction for 5 min. Hundred micromolar NMDA was added to initiate the swimming motor network [17] . GCaMP3-expressing cells were frame scanned at 200 Hz using the resonance scanner of a Leica SP5 confocal microscope. Confocal software was used to measure relative fluorescence intensity changes and kinetics of induced Ca 2+ transients. Immunolabelling Whole mount embryos were immunolabelled as described previously [26] . For labelling dissociated skeletal muscle fibres, 48 hpf embryos were incubated in collagenase type II (3.125 mg ml −1 in CO 2 -independent medium) at 20 °C for 1.5 h with the muscle fibres triturated every 30 min. Fibres were spun at 380 g for 5 min, supernatant removed and fibres resuspended and allowed to settle on polyornithine-coated coverslips. Fibres were washed then fixed. Dissociated muscles were labelled using 0.25% detergent in the incubation solutions containing the following primary antibodies/toxin: 1/200 dilution of anti-RyR (34C IgG1, Sigma); 1/200 anti-DHPR α1 (1A IgG1, Affinity BioReagents); 1/10 bungarotoxin-Alexa594 (Invitrogen); 1/500 anti-SV2; 1/200 anti-α actinin; and 1/200 anti-dystrophin (all from Iowa Hybridoma Bank). In some cases nuclei were labelled with 0.1% 4′,6-diamidino-2-phenylindole. Positional cloning of stac3 To identify the gene mutated in stac3 mi34 mutants, the mutation was meiotically mapped to PCR-scorable, polymorphic CA repeats as described previously [45] by scoring 2009 mutant embryos derived from appropriate mapping crosses. Flanking markers were identified located on linkage group 9; z1830 that was 0.21 cM north of stac3 mi34 and z1663 that was 1.24 cM south. Analysis of the zebrafish genome database ( http://www.sanger.ac.uk/resources/zebrafish/ ) revealed that z1830 was located in a small contig of assembled sequence (Scaffold 450) from the zV5 assembly of the sequenced genome that contained the pcbp2 gene. A new marker (zh1) located in pcbp2 mapped 0.11 cM north of stac3 mi34 . A sequenced 156-kb BAC (CR848672) that contained pcbp2 was identified and analysed for potential genes with the gene prediction program, GENSCAN ( http://genes.mit.edu/GENSCAN.html ), and BLASTing predicted genes against the NCBI database ( http://www.ncbi.nlm.nih.gov/BLAST ). These were pcbp2, kif5a, arp5 and a gene similar to stac . New markers, zh34 in kif5a (0.04 cM north), zh16 in arp5 (0.04 cM south) and zh31 in the stac -like gene (no recombinants), were identified. The stac -like cDNA from wt and mutant embryos were isolated and sequenced, and the mutant cDNA contained an insertion that included an in-frame stop codon. Analysis of genomic sequences determined that the stac3 mi34 allele contained a missense mutation that transformed a splice donor site for the intron between exons 4 and 5 (GT to AT), which presumably lead to incorrect splicing and inclusion of the intron in the cDNA. Mutant rescue Rescue of stac3 mi34 behaviour was performed by subcloning zebrafish stac3 wt , stac3 mi34 , stac3 NAM or human STAC3 into pHSP70-EGFP [42] . Zebrafish stac3 NAM construct was generated by site-directed mutagenesis. Constructs (10 ng μl −1 ) were injected into one-cell stage progeny of stac3 mi34 carriers with a Nanoject II. At 48 hpf, stac3 mi34 mutant embryos were behaviourally identified and heat induced by switching them from water at 28.5 ° C to 37 ° C for 1 h. After heat induction, embryos were switched back to 28.5 ° C and assayed 3 and 24 h later. Embryos with ~10% or more skeletal muscle fibres expressing EGFP were used for behavioural assays. Responses of embryos to touch were video recorded and measured. For Ca 2+ imaging of Stac3 wt - or Stac NAM -expressing muscle fibres pHSP70:stac3 wt -mCherry and pHSP70:stac3 NAM -mCherry were generated along with α-actin:GCaMP3 . Embryos were injected with a 1:1 mixture of a stac3 construct and α-actin:GCaMP3 each at 10 ng μl −1 . After heat induction, embryos with skeletal muscle fibres expressing both constructs were selected for Ca 2+ imaging. Analysis of maternal transcripts by RT-PCR The start of midblastula transition and earliest zygotic transcription is at 3 hpf in zebrafish [34] . Fifty embryos at 2 and 3 hpf each were placed in Trizol, and RT-PCR was performed for stac3 and tuba1 ( tubulin α1 ), a house-keeping gene that is maternally expressed [46] . Exon-overlapping primer pairs shown below were designed to amplify ~200-bp fragments of cDNA from the 5′ (representing exons 3–6) or 3′ (exons 4–10) region of mature stac3 message. 5′ Primer pair (forward: 5′-GGACGACAACACTGTGTATTTTGTGTATG-3′; reverse: 5′-GAACCCAGGAGGTATTTTGCCGAAGCATCT-3′); 3′ primer pair (forward: 5′-ACGGATGATTGTTCTCAATAATAAGTTTGC-3′ reverse: 5′-CGCAACAGATGACAAGAACAAGAAGCAG-3′). Antisense MO knockdowns 4.6 nl of 400 μM solutions of translation-blocking antisense MO (GeneTools) or standard control MO were injected into recently fertilized embryos from crosses of stac3 mi34 carriers using a Nanoject II. The sequence of the antisense stac3 MO was: 5′-TCATATTGAGC CAT CAGTCCAGC-3′ with CAT corresponding the start ATG. For morphant rescue experiments, 10 ng μl −1 of α-actin:stac3 - egfp was coinjected along with the antisense MOs. Embryos were assayed for response to touch with forceps at 48 hpf and subsequently fixed and assayed with anti-Stac3. Polyclonal antiserum production and purification Full-length zebrafish Stac3 was expressed as a His–Sumo fusion protein in B21(DE3) cells (Invitrogen), and affinity-purified using Ni-NTA agarose. Protein was further purified by electrophoresis in a NuPAGE 4–12% SDS–polyacrylamide gel electrophoresis (SDS–PAGE) Bis-Tris Gel and subsequent excision of appropriate Coomassie-stained band. Rabbits were immunized with gel slices of purified fusion proteins. Antiserum was purified by passing through a Sulfolink column (Thermo) containing the immobilized fusion protein. Fragment of Stac3 that was bound by anti-Stac3 was identified as follows. Full-length stac3 cDNA and the fragment that encodes amino acids 1–63 were cloned in frame into pGADGT7 (Clontech), which contains an N-terminal HA tag and Gal4 activation domain. Each construct was transformed into Y2HGold Yeast using Yeastmaker Yeast Transformation system 2 (Clontech) and plated on appropriate auxotrophic media. Yeast was grown, collected and protein extracted with YPER yeast protein extraction reagent (Thermo). Protein samples were loaded for SDS–PAGE analysis, blotted onto nitrocellulose and probed separately with anti-HA or anti-Stac3. Western analysis and immunoprecipitation Fifty stac3 mi34 mutant and sibling embryos each were collected, lysed and the isolated protein loaded and separated by SDS–PAGE [22] . Anti-DHPR α1 was used for immunoblotting at 1:500, anti-pan-RyR at 1:2,000. Adult female fish were killed using 0.1% tricaine, skeletal muscle dissected on dry ice and total protein extracted. Protein lysate from an individual fish was immunoprecipitated using anti-DHPR α1 (1:100), or anti-pan-RyR (1:200) cross-linked with BS 3 (Thermo) to Protein G Dynabeads (Invitrogen). Generation of stable transgenic line α- Actin:stac3-gfp construct was injected at 20 ng μl −1 into the cytoplasm of embryos at the one-cell stage. Fish were raised to adulthood and germline founders identified by screening F1 progeny for GFP fluorescence. GFP-positive offspring were raised to establish the transgenic line. Mass spectrometry and data analysis Skeletal muscle lysates from 10 adult α- actin:stac3-gfp transgenic fish were pooled for immunoprecipitation with anti-GFP (Torrey Pines Biolabs Inc.) or normal mouse IgG. The pull-down fraction was separated using SDS–PAGE, and the fractions in the gel stained using Silver Stain Kit (Pierce). Thirteen bands appearing in the anti-GFP pull-down fraction lane but not in normal IgG pull-down lane were excised, washed with 25 mM ammonium bicarbonate followed by acetonitrile, reduced with 10 mM dithiothreitol at 60 °C followed by alkylation with 50 mM iodoacetamide at room temperature, and digested with trypsin at 37 °C for 4 h. Mass spectrometry was performed by the University of Michigan Proteomics and Peptide Synthesis Core using a nano LC/MS/MS with a Waters NanoAcquity HPLC system interfaced to a ThermoFisher LTQ Orbitrap Velos. Peptides were loaded on a trapping column and eluted over a 75-μm analytical column at 350 nl min −1 ; both columns were packed with Jupiter Proteo resin (Phenomenex). The mass spectrometer was operated in data-dependent mode, with MS performed in the Orbitrap at 60,000 FWHM resolution and MS/MS performed in the LTQ. The fifteen most abundant ions were selected for MS/MS. MS/MS samples were analysed using Mascot (Matrix Science, London). Mascot was set up to search the ipi.DANRE.v3.75.decoy database (74,790 entries). Mascot was searched with a fragment ion mass tolerance of 0.50 Da and a parent ion tolerance of 10.0 p.p.m. Carbamidomethyl of cysteine was specified in Mascot as a fixed modification. Scaffold (version Scaffold_3.1.2, Proteome Software Inc., Portland, OR) was used to validate MS/MS-based peptide and protein identifications. Peptides were identified at >95% probability and proteins were identified if they contained at least two identified peptides with each peptide identified in the protein at >95% probability. Peptide and protein probabilities were assigned by the Protein Prophet algorithm [47] . Proteins that contained similar peptides and could not be differentiated based on MS/MS analysis alone were grouped to satisfy the principles of parsimony. Molecular analysis of NAM The cohort of individuals with NAM was previously described [34] . NAM subjects were of Lumbee Indian descent with congenital muscle weakness who demonstrate two or more of the following phenotypic characteristics: myopathic facies, susceptibility to malignant hyperthermia, kyphoscoliosis and cleft palate. The probands were ascertained from the University of North Carolina at Chapel Hill Pediatric Genetics Clinic and from the Duke University Muscular Dystrophy Clinic. All data and samples were collected following informed consent of subjects; this study was approved by the Duke University Medical Center and the University of North Carolina Institutional Review Boards. DNA was extracted from whole blood using the Puregene system (Gentra Systems, Minneapolis, MN) and stored in the laboratory of the Duke Center for Human Genetics. Initially, each exon and the surrounding splicing regions of STAC3 were screened in three NAM patients and three related individuals through PCR amplification and automated Sanger sequencing. After identification of the NAM mutation in exon 10 of STAC3 , the entire cohort of available samples from NAM pedigrees was screened by exon amplification and sequencing for the mutation. In all, a total of 18 individuals from five Lumbee families were sequenced, as well as three unrelated unaffected Lumbee individuals. In addition, genomic DNA was screened from two neurologically normal control individuals (Coriell Institute NDPT006 and NDPT009) and from a collection of 111 adult subjects without evidence of neurological disease [48] . Electron microscopy Transmission electron microscopy was performed as previously described [7] , [49] . A minimum of three larvae per condition were examined. How to cite this article: Horstick, E. J. et al. Stac3 is a component of the excitation–contraction coupling machinery and mutated in Native American myopathy. Nat. Commun. 4:1952 doi: 10.1038/ncomms2952 (2013).